Anti-ghrelin immunoglobulins modulate ghrelin stability and its orexigenic effect in obese mice and humans Obese individuals often have increased appetite despite normal plasma levels of the main orexigenic hormone ghrelin. Here we show that ghrelin degradation in the plasma is inhibited by ghrelin-reactive IgG immunoglobulins, which display increased binding affinity to ghrelin in obese patients and mice. Co-administration of ghrelin together with IgG from obese individuals, but not with IgG from anorectic or control patients, increases food intake in rats. Similarly, chronic injections of ghrelin together with IgG from ob/ob mice increase food intake, meal frequency and total lean body mass of mice. These data reveal that in both obese humans and mice, IgG with increased affinity for ghrelin enhances ghrelin’s orexigenic effect, which may contribute to increased appetite and overeating. Obesity is commonly accompanied by increased hunger and food intake [1] . However, the plasma concentrations of ghrelin, the principal hunger hormone [2] , are not elevated [3] , [4] . This indicates that in obesity ghrelin may transmit even more powerful hunger signals to the central circuitries regulating appetite [5] , [6] . In fact, ghrelin administration has been shown to stimulate food intake more efficiently in obese than in lean humans [7] but the underlying mechanisms remain unknown. Ghrelin is secreted by the stomach as an acylated bioactive peptide [8] that degrades to des-acyl-ghrelin [9] having no orexigenic effects [10] . Earlier studies assaying total ghrelin in plasma have reported lower levels in obese subjects [3] , but as it was later clarified, this decrease might be due to the low levels of des-acyl-ghrelin, whereas acyl-ghrelin remains normal [4] , [11] suggesting decreased degradation of acyl-ghrelin in the obese. On the contrary, patients with anorexia nervosa (AN) display elevated plasma levels of both total [12] and acylated ghrelin [13] , indicating increased ghrelin production. Recently, ghrelin-reactive immunoglobulins (Ig), that is, autoantibodies (autoAbs), have been identified in healthy subjects [14] and in AN patients [15] . Furthermore, studies in rodents showed that gastric electrical stimulation of ghrelin secretion [16] leads to simultaneous increase of ghrelin-reactive IgG [17] , and that raising antibodies against ghrelin may lead to decreased body weight in immunized animals [18] . Consequently, it is possible that plasma ghrelin may be bound to naturally present ghrelin-reactive IgG and that changes of properties of such IgG may influence the biological activity of circulating ghrelin, including increasing the hormone’s orexigenic effect in obesity. In the present work, we determine that biologically available ghrelin in human plasma is bound to IgG, which protects it from degradation. Using surface plasmon resonance (SPR) technology [19] , we characterize the affinity kinetics between plasma IgG and ghrelin in obese subjects and leptin-deficient obese ob/ob mice [20] known for their hyperphagia [21] , revealing increased affinity of anti-ghrelin IgG in both obese mice and humans. We also show that IgG extracted from plasma of obese humans or ob/ob mice enhance ghrelin-induced feeding in rodents, supporting the involvement of ghrelin-reactive immunoglobulins in increased appetite and overeating in obesity. Ghrelin concentrations in patients and controls Plasma ghrelin and des-acyl ghrelin concentrations were determined in plasma acidified for the preservation of ghrelin from venous blood samples taken at 8:00 after overnight fast in patients with hyperphagic obesity ( n =14, body mass index (BMI)±s.e.m., 31.08±1.56 kg m −2 ), restrictive AN ( n =12, BMI±s.e.m. 13.33±0.38 kg m −2 ) and healthy lean controls ( n =14, BMI±s.e.m., 20.92±0.48 kg m −2 ) (all females; age±s.e.m., 23.14±1.08 years, 21.42±1.9 years and 18.86±1.14 years, respectively). As expected, concentrations of both ghrelin and des-acyl ghrelin were elevated in AN patients ( Fig. 1a,b ), whereas ghrelin and des-acyl ghrelin in the obese did not differ significantly from that in controls ( Fig. 1a,b ). To determine whether plasma ghrelin was bound to circulating IgG, we measured concentrations of both ghrelin and des-acyl ghrelin in the eluates of IgG extracted from human plasma. We found that both ghrelin and des-acyl ghrelin bound to IgG were well detectable in all three study groups, although relatively more ghrelin than des acyl-ghrelin was found in the IgG-bound form ( Fig. 1c,d ). Ghrelin and des-acyl ghrelin concentrations were then assayed in the IgG-deprived plasma effluents, revealing increased levels of IgG unbound ghrelin in obese patients versus controls ( Fig. 1c ), whereas IgG unbound des-acyl ghrelin was higher only in AN patients ( Fig. 1d ). The cumulative ghrelin concentrations resulting from the sum of ghrelin measured in the IgG-bound and unbound fractions of the same plasma samples were increased in both obese and AN patients as compared with controls ( Fig. 1c ), whereas cumulative des-acyl ghrelin was increased only in AN patients ( Fig. 1d ). The ratios of ghrelin to des-acyl ghrelin did not significantly differ among the groups ( Fig. 1e ). 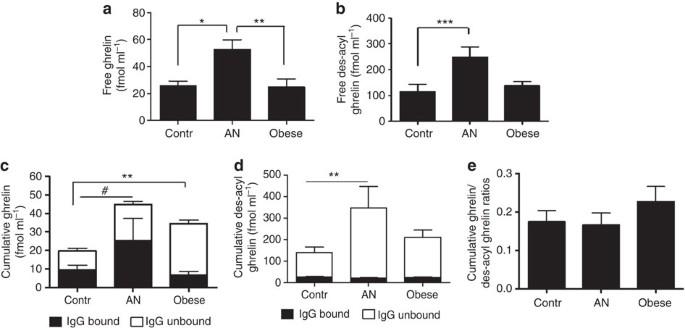Figure 1: Ghrelin and des-acyl ghrelin concentrations in humans. Plasma concentrations of ghrelin (a) and des-acyl ghrelin (b) before IgG extraction. Ghrelin (c) and des-acyl ghrelin (d) bound to the plasma-extracted IgG or IgG unbound assayed in IgG-deprived effluents of the same plasma samples are shown in the same bar as cumulative ghrelin concentrations for which statistical analysis is presented. Ratios of cumulative plasma concentrations between ghrelin and des-acyl ghrelin (e). (a) Kruskal–Wallis (K–W) test,P=0,002, Dunn’s *P<0.05, **P<0.01; (b) K–W test,P=0.0008, Dunn’s ***P<0.001; (c) K–W test,P=0.001, Dunn’s **P<0.01, Mann–Whitney test#P<0.05; (d) K–W (M-W) test,P=0,009, Dunn’s **P<0.01. (Contr.n=14, ANn=12 and obesen=14, error bars, s.e.m.). Figure 1: Ghrelin and des-acyl ghrelin concentrations in humans. Plasma concentrations of ghrelin ( a ) and des-acyl ghrelin ( b ) before IgG extraction. Ghrelin ( c ) and des-acyl ghrelin ( d ) bound to the plasma-extracted IgG or IgG unbound assayed in IgG-deprived effluents of the same plasma samples are shown in the same bar as cumulative ghrelin concentrations for which statistical analysis is presented. Ratios of cumulative plasma concentrations between ghrelin and des-acyl ghrelin ( e ). ( a ) Kruskal–Wallis (K–W) test, P =0,002, Dunn’s * P <0.05, ** P <0.01; ( b ) K–W test, P =0.0008, Dunn’s *** P <0.001; ( c ) K–W test, P =0.001, Dunn’s ** P <0.01, Mann–Whitney test # P <0.05; ( d ) K–W (M-W) test, P =0,009, Dunn’s ** P <0.01. (Contr. n =14, AN n =12 and obese n =14, error bars, s.e.m.). Full size image Anti-ghrelin IgG in patients and controls Next, to determine plasma levels of ghrelin-reactive IgG, we used enzyme-linked immunosorbent assay (ELISA). We found that the plasma levels of ghrelin-reactive IgG were similar in all three groups ( Fig. 2a ) but total IgG concentrations assayed by immunonephelometry were slightly lower in obese patients ( Fig. 2b ). As a specificity control, we also confirmed that detection of ghrelin-reactive IgG in ELISA was inhibited by preincubation of plasma with 10 −6 M ghrelin in both controls and obese, but it was ineffective in AN patients ( Fig. 2c–e ). 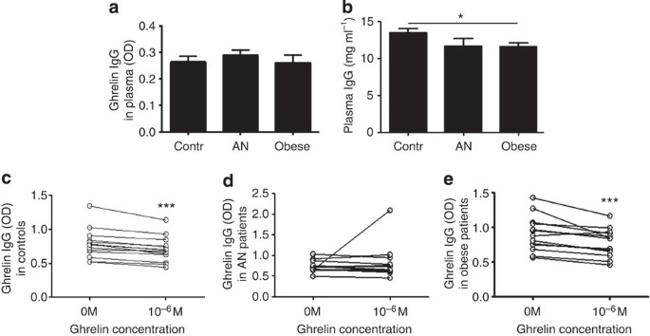Figure 2: Ghrelin-reactive IgG and total IgG in humans. Plasma levels of ghrelin-reactive IgG (a). Plasma concentrations of total IgG (b) measured by the nephelometry. Plasma levels in optical density (OD) of ELISA of ghrelin-reactive IgG before and after absorptions of plasma with 10−6M ghrelin in control subjects (c), AN patients (d) and obese (e). Absorption was efficient in controls and the obese but not in AN patients, probably due to increased dissociation properties of some AN patients’ IgG (Fig. 4f). (b) Student’st-test *P<0.05; (c,e) Pairedt-tests, ***P<0.001. (Contr.n=14, ANn=12 and obesen=14, error bars, s.e.m.). Figure 2: Ghrelin-reactive IgG and total IgG in humans. Plasma levels of ghrelin-reactive IgG ( a ). Plasma concentrations of total IgG ( b ) measured by the nephelometry. Plasma levels in optical density (OD) of ELISA of ghrelin-reactive IgG before and after absorptions of plasma with 10 −6 M ghrelin in control subjects ( c ), AN patients ( d ) and obese ( e ). Absorption was efficient in controls and the obese but not in AN patients, probably due to increased dissociation properties of some AN patients’ IgG ( Fig. 4f ). ( b ) Student’s t -test * P <0.05; ( c , e ) Paired t -tests, *** P <0.001. (Contr. n =14, AN n =12 and obese n =14, error bars, s.e.m.). Full size image The ability of a protein to act as a carrier for a small molecule depends on the specificity and reversibility of binding as determined by their affinity kinetics. In this study, we used SPR technology to determine affinity kinetics between ghrelin and IgG purified from the plasma of obese, AN or control subjects after plasma acidification and peptide extraction. By comparing the binding of each study subject’s IgG (0.5 mg ml −1 at flow speed of 5 μl min −1 ) to ghrelin, we found different dynamics of association and dissociation, resulting in an overall reduced SPR response in the obese as compared with controls and AN patients ( Fig. 3a ). A decrease in mean SPR resonance units (RU) values in obese was particularly evident at the end of association and was less pronounced after dissociation ( Fig. 3b,c ), indicating slower dissociation. 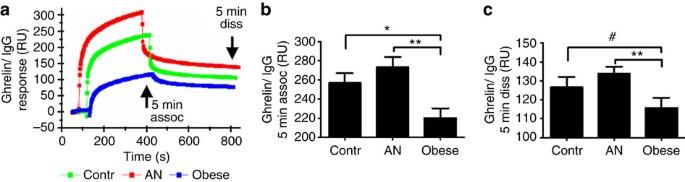Figure 3: Affinity binding between human ghrelin and IgG assayed by SPR. Representative SPR sensorgrams (a) of association and dissociation to ghrelin of IgG from obese (blue), controls (green) and AN patients (red) after single injection of 0.5 mg ml−1of IgG with low flow speed of 5 μl min−1. Mean SPR response in RU between three study groups 5 min after association (b) and 5 min after dissociation (c) as indicated by arrows in (a). (b) ANOVA,P=0.002, Tukey’s **P<0.01, *P<0.05; (c) K–W test,P=0.009, Dunn’s **P<0.01, M-W test,#P<0.05. (Contr.n=14, ANn=12 and obesen=14, error bars, s.e.m.). Figure 3: Affinity binding between human ghrelin and IgG assayed by SPR. Representative SPR sensorgrams ( a ) of association and dissociation to ghrelin of IgG from obese (blue), controls (green) and AN patients (red) after single injection of 0.5 mg ml −1 of IgG with low flow speed of 5 μl min −1 . Mean SPR response in RU between three study groups 5 min after association ( b ) and 5 min after dissociation ( c ) as indicated by arrows in ( a ). ( b ) ANOVA, P =0.002, Tukey’s ** P <0.01, * P <0.05; ( c ) K–W test, P =0.009, Dunn’s ** P <0.01, M-W test, # P <0.05. (Contr. n =14, AN n =12 and obese n =14, error bars, s.e.m.). Full size image Next, the affinity kinetics were analysed for each study subject using five consecutive IgG dilutions (from 0.5 to 0.03 mg ml −1 at flow speed of 30 μl min −1 ) and the 1:1 Langmuir’s fit model ( Fig. 4a–c ). In all study subjects, we found that the equilibrium dissociation constant KD values of ghrelin-reactive IgG were in the micromolar range between 10 −6 M and 10 −7 M. However, the mean KD, which is an inverse measure of affinity, was significantly lower in obese subjects than in controls (by a factor of 1.2) and than in AN patients (by a factor of 2.5) ( Fig. 4d ). This increase in affinity was mainly due to higher association rates (small K a values) in obese versus controls (by a factor of 3) ( Fig. 4e ), as mean dissociation rates (small K d values) in the obese were not significantly different from that in controls ( Fig. 4f ). In contrast, increased mean small K d values characterized IgG from AN patients ( Fig. 4f ). 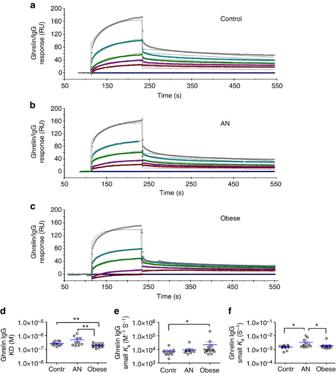Figure 4: Affinity kinetics between human ghrelin and IgG assayed by SPR. Affinity kinetics were analysed by the Langmuir’s 1:1 model fit on five serial dilutions of IgG from 0.5 mg ml−1and flow speed of 30 μl min−1. Representative examples of curve fits for the affinity kinetic analysis of a control subject (a), AN (b) and obese (c) patients. The affinity kinetics parameters of the given examples are the following: (a) smallka(±s.e.m.), 9.17 × 103±1.09 × 102M−1s−1, smallKd(±s.e.m.), 1.37 × 10−3±3.14 × 10−5s−1, KD, 1.50 × 10−7M,χ221.1; (b) smallKa(±s.e.m.), 8.76 × 103±1.17 × 102M−1s−1, smallKd(±s.e.m.), 1.78 × 10−3±3.52 × 10−5s−1, KD, 2.03 × 10−7M,χ213.7 and (c) smallKa(±s.e.m.), 1.71 × 104±2.53 × 102M−1s−1, smallKd(±s.e.m.), 1.77 × 10−3±3.98 × 10−5s−1, KD, 1.04 × 10−7M,χ212.3. Affinity for ghrelin of IgG in obese patients was increased compared to controls and AN patients as represented by lower meanKDvalues in obese (d). Association (Ka) and dissociation (Kd) rates are shown in (e) and (f), respectively. (d) K–W test,P=0,004, Dunn’s **P<0.01 AN versus obese, Student’st-test **P<0.01 controls versus obese; (e) K–W test,P=0.03, Dunn’s *P<0.05; (f) K–W test,P=0,034, Dunn’s *P<0.05 controls versus AN, M–W test, *P<0.05 AN versus obese. (Contr.n=14, ANn=12 and obesen=14, error bars, s.e.m.). Figure 4: Affinity kinetics between human ghrelin and IgG assayed by SPR. Affinity kinetics were analysed by the Langmuir’s 1:1 model fit on five serial dilutions of IgG from 0.5 mg ml −1 and flow speed of 30 μl min −1 . Representative examples of curve fits for the affinity kinetic analysis of a control subject ( a ), AN ( b ) and obese ( c ) patients. The affinity kinetics parameters of the given examples are the following: ( a ) small k a (±s.e.m. ), 9.17 × 10 3 ±1.09 × 10 2 M −1 s −1 , small K d (±s.e.m. ), 1.37 × 10 −3 ±3.14 × 10 −5 s −1 , KD, 1.50 × 10 −7 M, χ 2 21.1; ( b ) small K a (±s.e.m. ), 8.76 × 10 3 ±1.17 × 10 2 M −1 s −1 , small K d (±s.e.m. ), 1.78 × 10 −3 ±3.52 × 10 −5 s −1 , KD, 2.03 × 10 −7 M, χ 2 13.7 and ( c ) small K a (±s.e.m. ), 1.71 × 10 4 ±2.53 × 10 2 M −1 s −1 , small K d (±s.e.m. ), 1.77 × 10 −3 ±3.98 × 10 −5 s −1 , KD, 1.04 × 10 −7 M, χ 2 12.3. Affinity for ghrelin of IgG in obese patients was increased compared to controls and AN patients as represented by lower mean K D values in obese ( d ). Association ( K a ) and dissociation ( K d ) rates are shown in ( e ) and ( f ), respectively. ( d ) K–W test, P =0,004, Dunn’s ** P <0.01 AN versus obese, Student’s t -test ** P <0.01 controls versus obese; ( e ) K–W test, P =0.03, Dunn’s * P <0.05; ( f ) K–W test, P =0,034, Dunn’s * P <0.05 controls versus AN, M–W test, * P <0.05 AN versus obese. (Contr. n =14, AN n =12 and obese n =14, error bars, s.e.m.). Full size image We also analysed plasma levels and affinity kinetics of patients’ and controls’ IgG to bind des-acyl ghrelin, which showed no significant differences among the groups for either of their plasma levels ( Fig. 5a ) or parameters of affinity kinetics, with KD detected in the micromolar range ( Fig. 5b–d ). 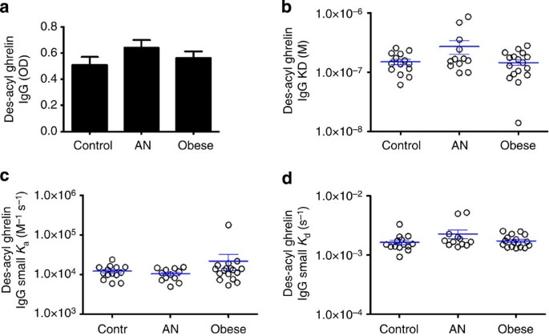Figure 5: Anti-des-acyl ghrelin IgG in humans. Plasma levels of des-acyl ghrelin-reactive IgG (a). Affinity kinetics between human des-acyl ghrelin and IgG showing: dissociation equilibrium constants (KD) (b), association rates (smallKa) (c) and dissociation rates (smallKd) (d). (Contr.n=14, ANn=12 and obesen=14, error bars, s.e.m.). Figure 5: Anti-des-acyl ghrelin IgG in humans. Plasma levels of des-acyl ghrelin-reactive IgG ( a ). Affinity kinetics between human des-acyl ghrelin and IgG showing: dissociation equilibrium constants (KD) ( b ), association rates (small K a ) ( c ) and dissociation rates (small K d ) ( d ). (Contr. n =14, AN n =12 and obese n =14, error bars, s.e.m.). Full size image Obese patients IgG enhance ghrelin orexigenic effects To determine whether IgG may modulate the orexigenic effects of ghrelin, we injected intraperitoneally in free-feeding rats ghrelin alone or together with human IgG characterized by different affinities for ghrelin. We used six IgG with the lowest RU values (increased affinity) from obese, six IgG with the highest RU (low affinity) from AN patients and six IgG that were most similar to the mean RU values in the control group. As we studied the interaction of human ghrelin with human autoAbs, we also used human ghrelin in the rat study. As it differs from rat ghrelin by two amino acids [2] , we first analysed the effect of human ghrelin on food intake in rats. We found that 3 nmol but not 1 nmol of human ghrelin increased 30-min food intake in rats, but it was less potent than rat ghrelin ( Fig. 6a,b ). Nevertheless, we selected the 1 nmol dose of human ghrelin for the co-administration experiment aiming at better distinguishing potential modulatory effects of IgG on ghrelin-induced food intake; in fact, 1 nmol of rat ghrelin was previously identified as the smallest dose stimulating food intake in satiated rats [22] . After co-administration of 1 nmol of human ghrelin with 1 nmol of IgG from obese, AN patients or controls, we found that only rats receiving the combination with IgG from obese displayed increased food intake as compared with the other groups ( Fig. 6c ). This orexigenic effect was acute and gradually disappeared by 12 h after injection ( Fig. 6d ). The enhanced feeding effect associated with obese IgG was linked to their co-administration with ghrelin, as injection of 1 nmol of the same IgG alone had no effects on food intake in free-feeding rats at 30 min or later ( Fig. 6e,f ). 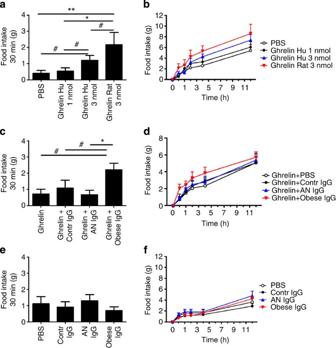Figure 6: Acute effects of human IgG on ghrelin-induced food intake in rats. Comparison of orexigenic effects of human (Hu) ghrelin and rat ghrelin in satiated rats (a,b). Higher 30 min food intake in free-fed rats was induced by co-administration of human ghrelin (1 nmol), together with IgG purified from plasma of obese (1 nmol) (c,d), which alone did not significantly change food intake as a shown in (e,f). (a) ANOVA,P=0,005, Tukey’s **P<0.01, *P<0.05, Student’st-tests#P<0.05; (c) ANOVA,P=0,031, Tukey’s *P<0.05, Student’st-tests#P<0.05. (n=6, error bars, s.e.m.). Figure 6: Acute effects of human IgG on ghrelin-induced food intake in rats. Comparison of orexigenic effects of human (Hu) ghrelin and rat ghrelin in satiated rats ( a , b ). Higher 30 min food intake in free-fed rats was induced by co-administration of human ghrelin (1 nmol), together with IgG purified from plasma of obese (1 nmol) ( c , d ), which alone did not significantly change food intake as a shown in ( e , f ). ( a ) ANOVA, P =0,005, Tukey’s ** P <0.01, * P <0.05, Student’s t -tests # P <0.05; ( c ) ANOVA, P =0,031, Tukey’s * P <0.05, Student’s t -tests # P <0.05. ( n =6, error bars, s.e.m.). Full size image Patients’ and controls’ IgG protect ghrelin from degradation To test whether IgG might protect ghrelin from degradation by plasma-hydrolysing enzymes, we studied in vitro stability of 30 fmol ml −1 of ghrelin, which is in the range of physiological plasma ghrelin levels, after its incubation for 2 h at 37 °C in the IgG-deprived plasma effluents alone or together with 1 nmol of IgG extracted from the same plasma samples. We found that after incubation of ghrelin together with IgG from either controls, AN or obese patients, most of the initially added ghrelin could be detected in the incubation milieu without significant differences between the groups ( Fig. 7a ). However, when ghrelin was incubated alone, its concentration was strongly decreased, indicating its rapid degradation ( Fig. 7a ). Furthermore, the efficiency of protection of ghrelin against degradation was more pronounced with IgG from the obese group ( Fig. 7b ). 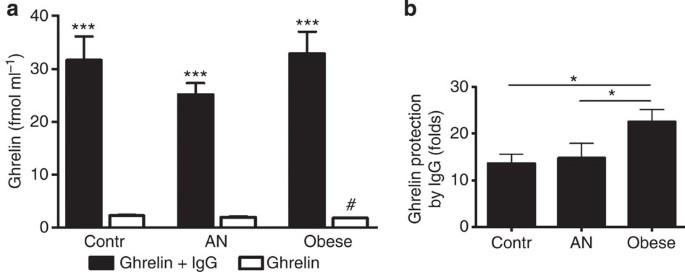Figure 7: Ghrelin degradation is reducedin vitroby human IgG. Ghrelin concentrations after incubation of ghrelin (30 fmol ml−1) in the IgG-deprived plasma effluents for 2 h at 37°C with and without human IgG (a). Estimation of ghrelin protection efficiency from degradation by the ratios of ghrelin concentrations measured after incubations of ghrelin with IgG versus ghrelin alone (b). (a) M–W tests ***P<0.001, Student’st-tests#P<0.05 versus controls; (b) Student’st-tests *P<0.05. (n=6, error bars, s.e.m.). Figure 7: Ghrelin degradation is reduced in vitro by human IgG. Ghrelin concentrations after incubation of ghrelin (30 fmol ml −1 ) in the IgG-deprived plasma effluents for 2 h at 37°C with and without human IgG ( a ). Estimation of ghrelin protection efficiency from degradation by the ratios of ghrelin concentrations measured after incubations of ghrelin with IgG versus ghrelin alone ( b ). ( a ) M–W tests *** P <0.001, Student’s t -tests # P <0.05 versus controls; ( b ) Student’s t -tests * P <0.05. ( n =6, error bars, s.e.m.). Full size image Ghrelin and anti-ghrelin IgG in ob/ob and lean mice To further analyse the relevance of ghrelin-reactive IgG to food intake and obesity we studied their properties in 2-month-old male obese ob/ob mice (body weight ±s.d., 51.4±1.8 g, n =11) as compared with male wild-type lean mice (body weight ±s.d., 25.6±1.8 g, n =12) of the same age and the same C57Bl6 genetic background. In vivo analysis of body composition showed increased total fat mass in ob/ob versus lean mice (27.6±1.8 g ±s.d., versus 2.9±1.6 g ±s.d., respectively, Student’s t -test P <0.0001) but total lean mass was not significantly different (21.4±1.4 g ±s.d., versus 20.4±1.4 g ±s.d., respectively, Student’s t -test P =0.07). Plasma concentrations of both ghrelin and des-acyl ghrelin were slightly lower in ob/ob than in lean mice ( Fig. 8a,b ), but the ratios of ghrelin to des-acyl ghrelin did not differ between the two groups ( Fig. 8c ). Plasma levels of ghrelin-reactive IgG were also slightly lower in ob/ob than in lean mice ( Fig. 8d ). Levels of ghrelin-reactive IgG were also measured in tissues homogenates of the hypothalamus and liver, showing their presence at the detection limit with no significant differences between the groups ( Fig. 8e,f ), whereas in the stomach tissue ghrelin-reactive IgG were undetectable. 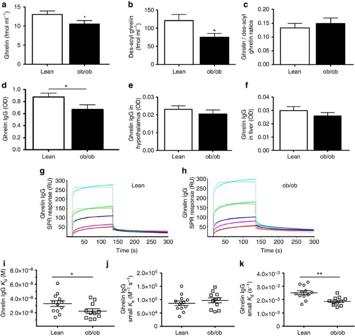Figure 8: Ghrelin and ghrelin-reactive IgG inob/oband lean mice. Plasma levels of ghrelin (a) and des-acyl ghrelin (b). Ghrelin to des-acyl ghrelin ratios (c). Plasma levels of ghrelin-reactive IgG (d). Tissue levels of ghrelin-reactive IgG in the hypothalamus (e) and liver (f). Affinity kinetics of plasma-extracted IgG and ghrelin as analysed by the SPR using the Langmuir’s 1:1 model fit. Representative examples of affinity kinetics of IgG for ghrelin in lean (g) and obese (h) mice with following parameters: (g) smallKa(±s.e.m.) 1.04 × 105±8.7 × 103M−1s−1, smallKd(±s.e.m.), 3.3 × 10−3±1.37 × 10−4s−1, KD, 3.18 × 10−8M,χ228,5 and (h) smallKa(±s.e.m.), 8.16 × 104±2.03 × 103M−1s−1, smallKd(±s.e.m.), 1.74 × 10−3±4.11 × 10−5s−1, KD, 2.13 × 10−8M,χ217.1. Dissociation equilibrium constants (KD) (i). Association rates (smallKa) (j). Dissociation rates (smallKd) (k). (a,b,d) Student’st-tests *P<0.05; (i,k) M–W tests *P<0.05, **P<0.01. (lean,n=12,ob/ob,n=11, error bars, s.e.m.). Figure 8: Ghrelin and ghrelin-reactive IgG in ob/ob and lean mice. Plasma levels of ghrelin ( a ) and des-acyl ghrelin ( b ). Ghrelin to des-acyl ghrelin ratios ( c ). Plasma levels of ghrelin-reactive IgG ( d ). Tissue levels of ghrelin-reactive IgG in the hypothalamus ( e ) and liver ( f ). Affinity kinetics of plasma-extracted IgG and ghrelin as analysed by the SPR using the Langmuir’s 1:1 model fit. Representative examples of affinity kinetics of IgG for ghrelin in lean ( g ) and obese ( h ) mice with following parameters: ( g ) small K a (±s.e.m.) 1.04 × 10 5 ±8.7 × 10 3 M −1 s −1 , small K d (±s.e.m. ), 3.3 × 10 −3 ±1.37 × 10 −4 s −1 , KD, 3.18 × 10 −8 M, χ 2 28,5 and ( h ) small K a (±s.e.m. ), 8.16 × 10 4 ±2.03 × 10 3 M −1 s −1 , small K d (±s.e.m. ), 1.74 × 10 −3 ±4.11 × 10 −5 s −1 , KD, 2.13 × 10 −8 M, χ 2 17.1. Dissociation equilibrium constants (KD) ( i ). Association rates (small K a ) ( j ). Dissociation rates (small K d ) ( k ). ( a , b , d ) Student’s t -tests * P <0.05; ( i , k ) M–W tests * P <0.05, ** P <0.01. (lean, n =12, ob/ob , n =11, error bars, s.e.m.). Full size image Affinity kinetics between plasma-extracted IgG and mouse ghrelin were analysed by SPR technology as used for characterizing human IgG described above ( Fig. 8g,h ). We found that IgG from ob/ob mice had increased affinities for ghrelin, manifested by lower KD values than in lean mice, which all remained in the 10 −8 M range ( Fig. 8i ). In contrast to ghrelin-reactive IgG in obese humans, this increase in affinity was due to lower dissociation rates ( Fig. 8k ), whereas association rates did not differ significantly between the groups ( Fig. 8j ). Obese mice IgG enhances ghrelin’s orexigenic effect To study the potential modulatory role of IgG in ghrelin-induced food intake in mice, mouse ghrelin was chronically injected in 1-month-old male lean C57Bl6 mice alone or in combination with IgG extracted from plasma of ob/ob or lean mice. For this purpose, two IgG pools were prepared from the IgG of six ob/ob and six lean mice characterized by low and high KD values, respectively, as determined by SPR. Mice received two daily intraperitoneal injections of ghrelin or ghrelin together with one of the IgG pools at the beginning of the light phase and before the onset of the dark phase for 2 weeks. Ghrelin doses were 0.1 nmol during the first 4 days and 1.0 nmol thereafter. The overall dynamics of body weight changes showed superior weight gain in mice receiving ghrelin with ob/ob IgG, although after 14 days of injections it still did not reach significance (day 15, Student’s t -test P =0.06, versus controls) ( Fig. 9a ). However, the body composition analysis at day 15 showed that total lean mass was increased in mice receiving ghrelin with ob/ob IgG ( Fig. 9b ). Surprisingly, percentage of body fat was not increased in this group and was even smaller than in mice receiving chronic injections of ghrelin alone ( Fig. 9c ). Daily mean food intake during the 14 days of injections was ~0.5 g higher in mice receiving ghrelin with ob/ob IgG than in controls and mice receiving ghrelin with lean IgG ( Fig. 9d ). The acute (30 min) enhancing effects of ob/ob IgG on ghrelin-induced feeding was visible already at the 0.1 nmol dose of ghrelin, although it was significant only after the evening but not morning injections ( Fig. 9e,f ). In contrast, with the dose of 1.0 nmol of ghrelin the acute IgG-enhancing effects were clear after the morning injections ( Fig. 9g ), whereas no further increase of the stimulatory effects of ghrelin were observed after the evening injections ( Fig. 9h ). The analysis of food intake according to the light/dark phases showed increased food intake in mice receiving 0.1 nmol of ghrelin with ob/ob IgG in dark but not in light phase ( Fig. 9i,j ), whereas the dose of 1.0 nmol increased food intake in light phase in all ghrelin-injected groups ( Fig. 9k ) and in mice co-injected with ob/ob IgG in the dark phase ( Fig. 9l ). The analysis of the feeding pattern showed that increased food intake in ghrelin plus ob/ob IgG-injected mice was due to increased meal number ( Fig. 9m ) while meal size was unchanged ( Fig. 9n ). 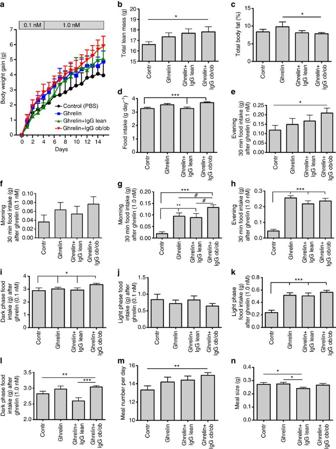Figure 9: Effects of chronic ghrelin administration in lean mice with or without IgG from lean or obese mice. Body weight gain during two daily injections of 0.1 nmol and 1.0 nmol of ghrelin alone or in combination with IgG from lean orob/obmice as compared to controls that received PBS (a). Body composition analysis at day 15 showing total lean mass (b) and percentage of body fat (c). Daily food intake during 14 days (d). Thirty-minute food intake after evening (e) and morning (f) injections of 0.1 nmol of ghrelin during 4 days. Thirty-minute food intake after morning (g) and evening (h) injections of 1.0 nmol of ghrelin during 10 days. Dark phase (i) and light phase (j) food intake after 0.1 nmol ghrelin injections during 4 days. Light phase (k) and dark phase (l) food intake after 1.0 nmol ghrelin injections during 10 days. Meal frequency (m) and meal size (n) during 14 days. (a) Two-way repeated measurements ANOVAP=0.24; (b,c,e,i,m,n) Student’st-tests *P<0.05,**P<0.01; (d,g,h,k,l) ANOVAP<0.0001, Tukey’s post tests **P<0.01, ***P<0.001, Student’st-tests#P<0.05. (n=6, error bars, s.e.m.). Figure 9: Effects of chronic ghrelin administration in lean mice with or without IgG from lean or obese mice. Body weight gain during two daily injections of 0.1 nmol and 1.0 nmol of ghrelin alone or in combination with IgG from lean or ob/ob mice as compared to controls that received PBS ( a ). Body composition analysis at day 15 showing total lean mass ( b ) and percentage of body fat ( c ). Daily food intake during 14 days ( d ). Thirty-minute food intake after evening ( e ) and morning ( f ) injections of 0.1 nmol of ghrelin during 4 days. Thirty-minute food intake after morning ( g ) and evening ( h ) injections of 1.0 nmol of ghrelin during 10 days. Dark phase ( i ) and light phase ( j ) food intake after 0.1 nmol ghrelin injections during 4 days. Light phase ( k ) and dark phase ( l ) food intake after 1.0 nmol ghrelin injections during 10 days. Meal frequency ( m ) and meal size ( n ) during 14 days. ( a ) Two-way repeated measurements ANOVA P =0.24; ( b , c , e , i , m , n ) Student’s t -tests * P <0.05,** P <0.01; ( d , g , h , k , l ) ANOVA P <0.0001, Tukey’s post tests ** P <0.01, *** P <0.001, Student’s t -tests # P <0.05. ( n =6, error bars, s.e.m.). Full size image Our work brings a new putative mechanism of ghrelin-mediated increase in appetite in obesity that may explain why ghrelin administration stimulates food intake more potently in obese than in normal-weight subjects, as previously reported [7] . We determined that plasma ghrelin-reactive IgG autoAbs can be responsible for this phenomenon, serving as carrier proteins that might enhance the bioactivity of endogenous or exogenous ghrelin. Although the existence of a ghrelin-binding protein could be suspected in analogy to some other peptide hormones [23] , the variable-affinity nature of IgG molecules makes them particularly interesting as potential modulators of ghrelin’s biological activities. In fact, ghrelin was readily detected in the protein G-purified IgG eluents but also in the remaining plasma effluents, indicating that in the circulation the hormone exists in both IgG-bound and unbound forms. Using these two measures to estimate the percentage of bound ghrelin might however not be accurate because a part of the initially IgG-bound ghrelin could flow into the effluents during the IgG linking to the column. In turn, the cumulative (bound and unbound) ghrelin concentrations measured in the plasma sample might be more informative. Indeed, in contrast to “free” ghrelin levels measured in native plasma, found to be similar between obese and controls in this study, we detected increased cumulative ghrelin concentrations in obese patients, suggesting that in the obese there is more IgG-bound ghrelin than in other groups and which was not detectable in whole plasma before IgG extraction. This might be related to the conformational changes of the IgG molecules upon its Fc fragment binding to protein G eventually resulting in release of ghrelin from the antigen-binding site [24] . As the Fc receptors are ubiquitously expressed in various immune cells, including brain microglia [25] , ghrelin–IgG complexes binding to Fc receptors might be one of the possible mechanisms of ghrelin release from the IgG that occurs in vivo . The biologically available IgG-bound fraction of circulating ghrelin, which was increased in obese patients, may hence contribute to ghrelin-mediated increased appetite in obesity. We also determined that obese patients had increased affinity of their IgG for ghrelin, which may underlie their ability to more efficiently bind and transport ghrelin as compared with IgG from controls and AN patients. Plasma levels of ghrelin-reactive IgG were not different between three study groups, further supporting that their different affinity kinetics, rather than levels, could be responsible for the enhanced orexigenic effects of ghrelin. Given that the increase in association rate was by factor 3 in IgG from obese, one may consider that while IgG from controls will bind one molecule of ghrelin, IgG from obese will bind three molecules. Additionally, a virtual absence of dissociations of ghrelin IgG in obese patients were visible after single injection of IgG at low flow speed, also indicating more stable ghrelin–IgG complexes. The micromolar range of the affinity of ghrelin-reactive IgG found in all study subjects is well positioned to mediate the peptide transport because it will not compete with the nano- to pico-molar affinity of interaction between ghrelin and its receptor [26] . Instead, ghrelin-reactive IgG might protect ghrelin from degradation by hydrolysing enzymes that deacylate ghrelin [9] , which generally display millimolar affinities for their substrates. Indeed, by an in vitro assay of ghrelin preservation from degradation by plasma enzymes we showed here that IgG protected ghrelin from degradation in all study groups but it was more pronounced by IgG from obese patients. Thus, a slight increase in affinity of ghrelin-reactive IgG in obesity might change these autoAbs to better ghrelin carriers/protectors, while not antagonizing ghrelin receptor binding. In agreement with these data, previous studies have also reported that micromolar affinity is a common feature of natural IgG autoAbs [27] . This is in contrast to high-affinity ghrelin-neutralizing antibodies, as produced by immunization, which were shown to reduce food intake after their peripheral administration in mice [28] , [29] . We did not find significant differences in the affinity of des-acyl ghrelin IgG between the controls and patients, which may indicate that ghrelin and des-acyl ghrelin do not bind to the same autoAbs and that rather ghrelin-reactive than des-acyl ghrelin-reactive IgG can modulate ghrelin’s orexigenic effects. As opposite to ghrelin and IgG affinity kinetics found in the obese, ghrelin-reactive IgG in AN patients displayed increased dissociation rates for ghrelin, indicating a tendency for decreased affinity for ghrelin, meaning that they will not be able to efficiently transport ghrelin and hence might diminish ghrelin’s orexigenic effects. Indeed, co-injections of ghrelin together with IgG from AN patients were not able to stimulate food intake in rats more than IgG from controls. In obese ob/ob mice, plasma IgG affinity for ghrelin was also increased mainly due to lower dissociation rates. The relevance of the differences of IgG properties between obese and lean mice to food intake and body weight was tested by chronic co-injections of IgG from ob/ob and lean mice together with ghrelin. Our results confirm the ability of IgG from obese mice to enhance ghrelin-stimulated food intake similar to the results seen in rats for IgG from obese humans. This effect was most obvious when measured acutely for 30 min after ghrelin injections and it was evident already at the smallest dose of ghrelin (0.1 nmol). Higher doses of ghrelin (1.0 nmol) strongly stimulated food intake in all groups of mice that received ghrelin in the evening. In contrast, the same dose of ghrelin injected in the morning produced higher food intake in mice receiving IgG from obese as compared with other groups. These data are in agreement with the previously reported differences of ghrelin stimulatory effects on food intake between light and dark phases [30] and may possibly contribute to increased overeating in obese animals in the light phase [31] . The mean daily food intake was also higher in mice that received ghrelin with ob/ob IgG, which was due to increased meal frequency but not meal size, pointing to increased hunger but not delayed satiation induced by this treatment, an observation in agreement with the accepted role of ghrelin to induce hunger [32] . Interestingly, while chronic injections of ghrelin with ob/ob IgG were associated with a tendency of increased body weight gain, the mice did not become fatter but rather gained more lean mass. Furthermore, mice injected with ghrelin alone showed higher total body fat than mice co-injected with ob/ob IgG. The fat tissue-inducing effects of chronic ghrelin administration in mice, not accompanied by increased food intake, have previously been documented [33] . The absence of adipogenic effect of ghrelin in mice co-injected with ob/ob IgG suggests that IgG induced more selective ghrelin actions on appetite controlling pathways and possibly also on the somatotropic axis. The mechanism of such selectivity needs further clarification. Our study also showed that not all obese subjects and obese mice had increased affinities of IgG for ghrelin, suggesting that such an increase is probably not the result of the obese phenotype or at least not its obligatory result. It means further that, although IgG would have a protective role for ghrelin against degradation by plasma enzymes in all subjects, it might be involved in enhancing ghrelin orexigenic effects only in those subjects and mice that display increased affinities for ghrelin. What makes humans and animals produce ghrelin-reactive IgG is presently unknown but the variation in their affinities in both obese and non-obese humans and animals suggests that there could be different antigenic stimulations possibly involving both ghrelin and ghrelin-like antigens such as those present in the gut microbiota for example, in proteins of Enterococcus fecalis bacteria [14] . In fact, germ-free rats display increased plasma levels of ghrelin-reactive IgG, indicating that they lack some microbial factors that would reduce an exaggerated ghrelin-reactive IgG production [14] . Hence, it is tempting to speculate that targeting ghrelin-reactive IgG via immuno-nutritional approaches may represent a new therapeutic target for appetite control in obesity and anorexia. In conclusion, our data reveal that plasma ghrelin is normally bound to circulating IgG, which may have a role as carriers for the hormone protecting it from degradation and further that IgG from obese patients seem to bind more ghrelin than IgG from non-obese subjects. We also show that IgG from both obese humans and ob/ob mice display elevated micromolar affinity for ghrelin, which may be responsible for an increased ability of these IgG to transport ghrelin and thus enhance its orexigenic and anabolic actions. It is likely that increased appetite and overeating observed in some obese humans and mice may be mediated at least partly by the circulating IgG enhancing the orexigenic effect of ghrelin, the main hunger peptide hormone. Study subjects Obese, AN patients and controls (all females; age±s.e.m., 23.14±1.08 years, 21.42±1.9 years and 18.86±1.14 years, respectively) were admitted to the Kagoshima University Hospital and gave written informed consent for study participation. AN patients were diagnosed according to the DSM-IV criteria [34] . The study was approved by the Ethical Committee of the Kagoshima University, Japan. Venous blood samples were collected into tubes containing ethylenediaminetetraacetic acid (EDTA, 1 mg ml −1 ), aprotinin (500 U ml −1 ) and 1 N HCl (1:10 vol). The plasma was separated by centrifugation at 4 °C and stored at −80 °C until assayed. Ghrelin and ghrelin-reactive IgG assays Ghrelin and des-acyl ghrelin concentrations in all experiments including human and mouse plasma were measured using EIA kits from Mitsubishi Chemical Med Corp, Tokyo, Japan. Plasma levels of IgG autoAbs reacting with ghrelin and des-acyl ghrelin were measured using ELISA according a published protocol [35] . For specificity controls of ghrelin-reactive IgG, prior to ELISA, human plasma samples were preincubated overnight at 4 o C with ghrelin diluted at 10 −6 M. Concentrations of plasma total IgG were assayed by immunonephelometry using specific antibodies (Siemens, Germany) on a BNII nephelometer (Siemens). Total IgG were purified from human and mouse plasma samples via extraction of peptides from plasma globulins by plasma acidification and separation on C-18 SEP column (Phoenix Pharmaceuticals, Burlingame, CA, USA) followed by purification using Melon Gel Kit (Thermo Scientific, Pierce, Rockford, IL, USA). Purified IgG were lyophilized and then reconstituted in the HBS-EP buffer (GE Healthcare, Piscataway, NJ, USA). Affinity kinetics assay of IgG for ghrelin Affinity kinetics of human IgG autoAbs for ghrelin was determined by SPR on a BIAcore 1000 instrument (GE Healthcare). Ghrelin (Peptide institute, Inc.) was diluted to 0.5 mg ml −1 in 10 mM sodium acetate buffer (pH 5.0) (GE Healthcare) and was covalently coupled on the sensor chip CM5 (GE Healthcare), using the amine coupling kit (GE Healthcare). All the measurements were done on the same sensor chip. To compare relative binding response between IgG and ghrelin in obese, AN patients and controls, purified IgG were diluted in each sample to 0.5 mg ml −1 (3360, nM) in HBS-EP buffer (GE Healthcare) and 25 μl were injected (INJECT) into the flow conduit of BIAcore instrument with a flow speed of 5 μl min −1 at 25 °C. The values of RU of the sensorgram were recorded 5 min after association and in the end of dissociation 5 min after stopping the injection. All samples were analysed in a random order and alternating injections of IgG from controls, obese and AN patients. For the affinity kinetic analysis, a multi-cycle method was run with five serial dilutions of each patient and control IgG: 0.5, 0.25, 0.125, 0.625 and 0.03125 (mg ml −1 ) including a duplicate of 0.125 mg ml −1 and a blank (buffer only). During each cycle, 60 μl were injected (KINJECT) into the flow conduit of the BIAcore instrument with flow speed of 30 μl min −1 at 25 °C followed by 5 min of dissociation. Between injections of each sample, the binding surface was regenerated with 10 mM NaOH resulting in the return of the sensorgram to the same baseline. The affinity kinetic data were analysed using BiaEvaluation 4.1.1 programme (GE Healthcare). For fitting kinetic data, the Langmuir’s 1:1 model was used and the sample values were corrected by subtracting the blank values resulting from the injection of HBS-EP buffer. Affinity kinetics between patients’ and controls’ IgG and des-acyl ghrelin and between mouse IgG and ghrelin were analysed by SPR as described above but with human des-acyl ghrelin and mouse ghrelin (both from Peptide institute, Inc.), respectively, coupled to the CM5 chip (GE Healthcare). Acute food intake experiments in rats All animal care and experimentation were in accordance with guidelines established by the National Institutes of Health, USA and approved by the Normandy Ethical Committee for Animal Experimentation. Two-month-old male Sprague-Dawley rats ( n =24), body weight 200–250 g (Janvier Labs, Genest-Saint-Isle, France) were kept in holding cages (three rats per cage) in a fully equipped animal facility under regulated environmental conditions (22±1 °C, on a 12 h light–dark cycle with lights on at 7:30) for 1 week. Standard pelleted rodent chow (RM1 diet, SDS, UK) and drinking water were available ad libitum . Three days before experiments, the rats were transferred to individual metabolism cages (Tecniplast, Lyon France) where they were fed ad libitum with the same RM1 diet but in powdered form (SDS) and drinking water was always available. Rats were divided into four groups ( n =6) to achieve similar body weight. Three food intake experiments were performed with 4 days interval between each experiment. Intraperitoneal injections (300 μl) were done at 11:00 and immediately thereafter rats were returned to their metabolism cages, which contained a preweighed amount of food. Food intake was measured at 30 min, 1, 2, 4 and 12 h. In experiment 1 human ghrelin and rat ghrelin (Peptide institute, Inc.) were injected in free-fed satiated rats. Human ghrelin was injected with the doses of: 1 nmol or 3 nmol per rat; rat ghrelin was injected with the dose of 3 nmol per rat; the control group received PBS. In experiment 2, rats received injections of six different IgG purified from plasma of either obese, or AN or control subjects and control group received PBS. In experiment 3, rats received 1 nmol of IgG as in experiment 2 but this time together with 1 nmol of human ghrelin. Each rat injected with IgG received the same IgG as in the previous experiment. The control group that previously was injected with PBS received 1 nmol of human ghrelin only. In vitro ghrelin preservation assay Human ghrelin (150 nmol; Peptide institute, Inc.) was diluted in the PBS and added to IgG-deprived plasma effluents of obese and AN patients and controls resulting in its final concentration of 30 fmol ml −1 . Ghrelin was incubated in each plasma effluents alone or with 1 nmol of the same subject IgG in a rotating incubator for 2 h at 37 °C. Then, the incubation milieu was used for measuring ghrelin concentrations as described above. Ghrelin and anti-ghrelin IgG assays in ob/ob and lean mice Two-month-old C57Bl6 male obese ob/ob and wild-type lean mice were purchased from Janvier Labs and acclimated to the animal facility for 1 week. The body composition in awake mice was analysed using EchoMRI (EchoMRI, Houston, TX, USA) and then mice were killed by decapitation and trunk blood was collected into tubes containing EDTA (1 mg ml −1 ), aprotinin (500 U ml −1 ) and 1 N HCl (1:10 vol). The plasma was separated by centrifugation at 4 °C and stored at −80 °C until assayed for ghrelin, des-acyl ghrelin and ghrelin-reactive IgG. Entire hypothalamus and fragments of the liver and of the gastric fundus were collected and homogenized in PBS with the cocktail of protease and phosphatase inhibitors (Sigma) for ghrelin IgG assay. Total IgG were extracted from mouse plasma and analysed by the SPR as described above. Chronic food intake experiments in mice One-month-old wild-type male C57Bl6 mice ( n =32) were purchased from Janvier Labs and acclimated to the animal facility for 1 week with 12 h light–dark cycle, lights on at 7:00. Then, the mice were placed individually in the BioDAQ mouse cages (Research Diets, Inc., New Brunswick, NJ, USA), each equipped with an automatic feeding monitor. After 3 days of acclimation to the BioDAQ cages, mice were divided into four groups ( n =8), each receiving one of four different treatments consisting of two daily intraperitoneal injections at 10:00 and at 18:45. of either: (i) PBS, (ii) ghrelin alone, (iii) ghrelin with IgG extracted from lean C57Bl6 mice and (iv) ghrelin with IgG extracted from ob/ob mice. Mouse ghrelin (Peptide institute, Inc.) was injected at the dose of 0.1 nmol during the first 4 days and 1.0 nmol for next ten days. Two IgG pools were prepared from IgG of six ob/ob and six lean mice characterized by low and high KD vales, respectively, as measured by the SPR and 1 nmol of IgG was given at each injection. Food (SERLAB, Montataire France) and drinking water were available ad libitum and body weight was measured daily. Feeding data were continuously monitored for 14 days and analysed using the BioDAQ data viewer 2.3.07 (Research Diets). For the meal pattern analysis, the inter-meal interval was set at 300 s. After 14 days of injections, body composition in mice was analysed by the EchoMRI. Statistical analysis Data were analysed and the graphs were plotted using the GraphPad Prism 5.02 (GraphPad Software Inc., San Diego, CA, USA). Normality was evaluated by the Kolmogorov–Smirnov test. Group differences were analysed by the analysis of variance (ANOVA) or the non-parametric Kruskal–Wallis test with the Tukey’s or Dunn’s post tests, according to the normality results. Where appropriate, individual groups were additionally compared using the Student’s t -test or the Mann–Whitney test according to the normality results. Effects of absorptions were analysed using the paired t -test. Body weight gain in mice was analysed using the two-way repeated measurement ANOVA. Data are shown as means±s.e.m. and for all tests, P <0.05 was considered statistically significant. How to cite this article: Takagi, K. et al . Anti-ghrelin immunoglobulins modulate ghrelin stability and its orexigenic effect in obese mice and humans. Nat. Commun. 4:2685 doi: 10.1038/ncomms3685 (2013).